The nucleoporin MEL-28 promotes RanGTP-dependent γ-tubulin recruitment and microtubule nucleation in mitotic spindle formation The GTP-bound form of the Ran GTPase (RanGTP), produced around chromosomes, drives nuclear envelope and nuclear pore complex (NPC) re-assembly after mitosis. The nucleoporin MEL-28/ELYS binds chromatin in a RanGTP-regulated manner and acts to seed NPC assembly. Here we show that, upon mitotic NPC disassembly, MEL-28 dissociates from chromatin and re-localizes to spindle microtubules and kinetochores. MEL-28 directly binds microtubules in a RanGTP-regulated way via its C-terminal chromatin-binding domain. Using Xenopus egg extracts, we demonstrate that MEL-28 is essential for RanGTP-dependent microtubule nucleation and spindle assembly, independent of its function in NPC assembly. Specifically, MEL-28 interacts with the γ-tubulin ring complex and recruits it to microtubule nucleation sites. Our data identify MEL-28 as a RanGTP target that functions throughout the cell cycle. Its cell cycle-dependent binding to chromatin or microtubules discriminates MEL-28 functions in interphase and mitosis, and ensures that spindle assembly occurs only after NPC breakdown. Chromosomes mediate the assembly of the nuclear envelope and NPCs in interphase and spindle assembly in mitosis [1] . RanGTP is produced around chromatin [2] and plays a central role in both cell cycle stages. RanGTP binds to importin-α/β and dissociates nuclear localization signal (NLS)-containing proteins from importins [3] , [4] , [5] . In mitosis, liberated NLS proteins play distinct roles in spindle assembly around chromosomes [6] . To explore Ran-regulated spindle assembly factors, we previously purified and identified NLS-containing microtubule-associated proteins (MAPs) from Xenopus egg extracts [7] . These included the nucleoporin MEL-28 (maternal effect lethal-28)/ELYS (embryonic large molecule derived from yolk sac). MEL-28 is required for NPC assembly in human HeLa cells and Caenorhabditis elegans [8] , [9] , [10] . Further analysis using Xenopus egg extracts revealed that MEL-28 binds to chromatin in a RanGTP-dependent manner at early stages of NPC assembly [11] . MEL-28 interacts with the Nup107–160 complex (Nup for nucleoporin), an important building block of the NPC, and recruits the complex to chromatin. When NPCs disassemble in mitosis, MEL-28 partially localizes to kinetochores [8] , [9] , [10] . Its depletion from human cells or C. elegans embryos leads not only to nuclear pore defects in interphase but also to mitotic defects in chromosome condensation, kinetochore assembly, spindle assembly and chromosome segregation [8] , [9] , [10] . All these findings raise the question of whether MEL-28 affects mitosis directly or through its function in NPC assembly. Here we find that MEL-28 dissociates from mitotic chromatin and re-localizes to the spindle as a MAP, and it is directly required for spindle assembly. MEL-28 promotes RanGTP-dependent γ-tubulin recruitment and microtubule nucleation. Our data show that MEL-28 is a RanGTP target that drives NPC assembly as cells exit mitosis and spindle assembly as cells enter mitosis. 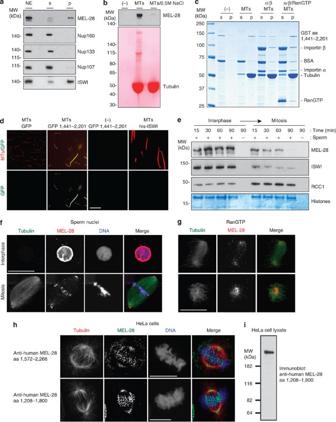Figure 1: MEL-28 is a RanGTP-dependent MAP that re-localizes from chromatin to the mitotic spindle. (a) HeLa nuclear extract (NE) was incubated with taxol-stabilized microtubules (MTs) and sedimented. Supernatant (s) and pellet (p) fractions were analysed by immunoblotting. (b) NE was incubated with or without MTs and with or without additional 0.5 M NaCl. After centrifugation, pellets were analysed by immunoblotting or Ponceau staining. (c) GST-fusedXenopusMEL-28 aa 1,441–2,201 was incubated with MTs in the presence or absence of importin-α, importin-β and RanGTP. After centrifugation, samples were analysed by Coomassie staining. (d) GFP, GFP-fused aa 1,441–2,201 or histidine-tagged ISWI were incubated with or without Cy3-labelled, taxol-stabilized MTs at RT for 10 min. Note that his-ISWI is a negative control that bundles MTs but does not show green signals. Bar, 20 μm. (e,f) Sperm nuclei inXenopusegg extract were cycled to interphase and then back to mitosis. (e) At indicated time points, chromatin was isolated and immunoblotted for MEL-28, ISWI and RCC1. Coomassie staining of the gel shows histones as an indicator of chromatin recovery. (f) Interphase nuclei and mitotic spindles were stained with aXenopusMEL-28 antibody (red) and Alexa488-labelled tubulin (green), as described in the methods. DNA was stained with Hoechst (blue). Bar, 20 μm. (g) CSF extract was incubated with RanGTP and Alexa488-tubulin (green). Ran-induced asters and spindles were stained with an MEL-28 antibody (red). Bars, 20 μm. (h) HeLa cells were pre-extracted with Triton X-100, fixed and stained with human MEL-28 antibodies against aa 1,572–2,266 (ref.11) or aa 1,208–1,800 fragments (green). Cells were also stained for α-tubulin (red) and DNA (blue). Bars, 10 μm. (i) Human MEL-28 antibody was generated in rabbits against recombinant aa 1,208–1,800. HeLa cell lysate was blotted with the antibody showing a monospecific signal at ~250 kD. MEL-28 is a Ran-dependent MAP that relocates to the spindle Our NLS-MAP purification [7] contained MEL-28 with a high score, similar to known RanGTP-regulated MAPs such as TPX2 ( Supplementary Table 1 ). Interestingly, Nup107 of the MEL-28-associated Nup107–160 complex (Nup160, Nup133, Nup107, Nup96, Nup85, Nup43, Nup37, Sec13 and Seh1, see Supplementary Table 1 ) was identified with a lower score, suggesting lower abundance. We examined the ability of MEL-28, included in HeLa nuclear extracts, to bind microtubules in a sedimentation assay. After sedimentation of taxol-stabilized microtubules, human MEL-28 was efficiently depleted from the extract and recovered in the pellet, similar to the nuclear MAP ISWI/SNF2H ( Fig. 1a ) [7] . In contrast, Nup107–160 components were not depleted ( Fig. 1a ) and were only detectable in the pellet when a 20-fold excess was probed ( Supplementary Fig. 1a ). MEL-28 was recovered in the pellet only in the presence of microtubules and under physiological salt concentration ( Fig. 1b ). Microtubule binding of MEL-28 was inhibited by recombinant importin-α and -β, but it was restored by further addition of RanGTP, similar to microtubule binding of ISWI (positive control) but not of ch-TOG (negative control) ( Supplementary Fig. 1b ). Figure 1: MEL-28 is a RanGTP-dependent MAP that re-localizes from chromatin to the mitotic spindle. ( a ) HeLa nuclear extract (NE) was incubated with taxol-stabilized microtubules (MTs) and sedimented. Supernatant (s) and pellet (p) fractions were analysed by immunoblotting. ( b ) NE was incubated with or without MTs and with or without additional 0.5 M NaCl. After centrifugation, pellets were analysed by immunoblotting or Ponceau staining. ( c ) GST-fused Xenopus MEL-28 aa 1,441–2,201 was incubated with MTs in the presence or absence of importin-α, importin-β and RanGTP. After centrifugation, samples were analysed by Coomassie staining. ( d ) GFP, GFP-fused aa 1,441–2,201 or histidine-tagged ISWI were incubated with or without Cy3-labelled, taxol-stabilized MTs at RT for 10 min. Note that his-ISWI is a negative control that bundles MTs but does not show green signals. Bar, 20 μm. ( e , f ) Sperm nuclei in Xenopus egg extract were cycled to interphase and then back to mitosis. ( e ) At indicated time points, chromatin was isolated and immunoblotted for MEL-28, ISWI and RCC1. Coomassie staining of the gel shows histones as an indicator of chromatin recovery. ( f ) Interphase nuclei and mitotic spindles were stained with a Xenopus MEL-28 antibody (red) and Alexa488-labelled tubulin (green), as described in the methods. DNA was stained with Hoechst (blue). Bar, 20 μm. ( g ) CSF extract was incubated with RanGTP and Alexa488-tubulin (green). Ran-induced asters and spindles were stained with an MEL-28 antibody (red). Bars, 20 μm. ( h ) HeLa cells were pre-extracted with Triton X-100, fixed and stained with human MEL-28 antibodies against aa 1,572–2,266 (ref. 11 ) or aa 1,208–1,800 fragments (green). Cells were also stained for α-tubulin (red) and DNA (blue). Bars, 10 μm. ( i ) Human MEL-28 antibody was generated in rabbits against recombinant aa 1,208–1,800. HeLa cell lysate was blotted with the antibody showing a monospecific signal at ~250 kD. Full size image ISWI binds to microtubules via the region containing chromatin-binding domains and an NLS [7] , which prompted us to test a potential direct microtubule-binding site of MEL-28 in its C terminus containing an AT-hook (AT-rich DNA-binding motif) and an NLS ( Supplementary Fig. 1c ) [12] . A MEL-28 C-terminal fragment comprising aa 1,441–2,201 bound to microtubules. Binding was inhibited by importin-α/β and restored by RanGTP ( Fig. 1c ). GFP-fused aa 1,441–2,201 bound along microtubules and bundled them ( Fig. 1d ). Strikingly, aa 1,602–2,120, lacking the AT-hook and NLS, did not bind to microtubules, whereas aa 1,993–2,201 bound ( Supplementary Fig. 1d ). Therefore, the C-terminal region containing AT-hook and NLS is the RanGTP-dependent microtubule-binding site of MEL-28. It has been reported previously that only a subpopulation of MEL-28 interacts with the Nup107–160 complex [11] . Consistently, when we immunodepleted MEL-28 from HeLa nuclear extracts, the Nup107–160 components were only partially depleted ( Supplementary Fig. 1e ). Importantly, microtubule binding of the remaining Nup107–160 components was inhibited in the sedimentation assay ( Supplementary Fig. 1e ), indicating that Nup107–160 complex binding to microtubules occurs via MEL-28. MEL-28 binds to microtubules via its chromatin-binding region, raising the question of how the distribution of MEL-28 between chromatin and microtubules is regulated during the cell cycle. By analysing chromatin re-isolated from cycling Xenopus egg extracts, we found that MEL-28 completely dissociates from chromatin on mitotic entry ( Fig. 1e ) [13] . In interphase egg extract, MEL-28 antibodies stained the rim and interior of in vitro- assembled nuclei ( Fig. 1f ) [8] , [11] . In the mitotic extract, we detected MEL-28 on kinetochores and spindle microtubules, with enrichment on spindle poles ( Fig. 1f ). Microtubule and pole localization was also observed in RanGTP-induced asters or spindle-like structures assembled in M-phase-arrested egg extracts in the absence of chromatin and kinetochores ( Fig. 1g ). MEL-28 has been shown to localize to kinetochores in mitotic cells [8] , [11] . We re-examined the localization of MEL-28 in HeLa cells. When soluble MEL-28 was extracted before fixation, residual MEL-28 was clearly detected around spindle poles, as well as on kinetochores ( Fig. 1h,i ). Therefore, spindle pole and kinetochore localization of MEL-28 is conserved in Xenopus and human cells. Independent MEL-28 functions in spindle and NPC assembly We next immunodepleted MEL-28 from M-phase-arrested Xenopus egg extracts and tested spindle formation around sperm nuclei ( Fig. 2a ) [14] . Nup107–160 components, as expected, were only partially depleted. 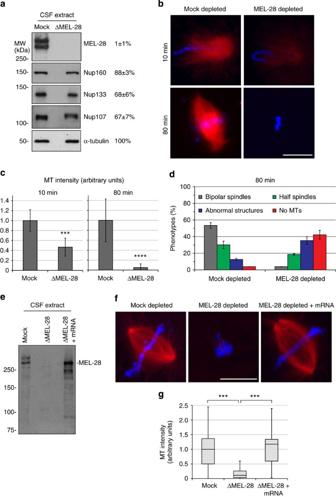Figure 2: MEL-28 is required for spindle assembly independently of its interphase function. (a) CSF extract was immunodepleted using rabbit IgG (mock) or aXenopusMEL-28 antibody, and analysed by immunoblotting. α-tubulin as a control protein was not depleted. Numbers (%, ±s.d. from three independent experiments) represent protein levels after MEL-28 depletion, quantified with non-saturated blots. (b–d) Spindle assembly around sperm nuclei was examined in control or MEL-28-depleted CSF extracts. At the indicated time point, aliquots were fixed and spun down on coverslips. (b) Representative images: blue, DNA; red, Cy3-labelled tubulin. (c) The microtubule (MT) intensity around sperm was quantified. We defined the MT intensity in control extracts as 1.n>20 structures. Error bars, s.d. (d) Quantification of spindle phenotypes over the total number of sperm counted.n>50 sperm. Error bars, s.d. from three experiments. (e–g) Control or MEL-28-depleted CSF extracts were incubated with or without mRNA encoding MEL-28 at 20 °C for 60 min, and spindle assembly was assayed as inb. (e) MEL-28 depletion and expression was analysed by immunoblotting. (f) Representative images. (g) Quantification of the MT intensity around sperm. Box-and-whisker plots show median (horizontal line), interquartile range (box) and maximum/minimum range (whiskers).n>30 structures from three independent experiments. ***P<0.001, ****P<0.0001 (Student’st-test, two-tailed). Bars, 20 μm. 10 min after incubation with sperm, MEL-28-depleted extracts did assemble microtubules but with significantly lower effectiveness than controls ( Fig 2b,c ). After 80 min, control extracts assembled bipolar spindles on sperm chromatin with ~50% frequency. In depleted extracts, the vast majority of sperm had no microtubules ( Fig. 2b–d ), indicating that initially generated microtubules were unstable. Importantly, when we expressed MEL-28 in depleted extracts using a corresponding mRNA, spindle assembly was fully restored yielding spindles with normal bipolarity and microtubule density ( Fig. 2e–g ). Figure 2: MEL-28 is required for spindle assembly independently of its interphase function. ( a ) CSF extract was immunodepleted using rabbit IgG (mock) or a Xenopus MEL-28 antibody, and analysed by immunoblotting. α-tubulin as a control protein was not depleted. Numbers (%, ±s.d. from three independent experiments) represent protein levels after MEL-28 depletion, quantified with non-saturated blots. ( b – d ) Spindle assembly around sperm nuclei was examined in control or MEL-28-depleted CSF extracts. At the indicated time point, aliquots were fixed and spun down on coverslips. ( b ) Representative images: blue, DNA; red, Cy3-labelled tubulin. ( c ) The microtubule (MT) intensity around sperm was quantified. We defined the MT intensity in control extracts as 1. n >20 structures. Error bars, s.d. ( d ) Quantification of spindle phenotypes over the total number of sperm counted. n >50 sperm. Error bars, s.d. from three experiments. ( e – g ) Control or MEL-28-depleted CSF extracts were incubated with or without mRNA encoding MEL-28 at 20 °C for 60 min, and spindle assembly was assayed as in b . ( e ) MEL-28 depletion and expression was analysed by immunoblotting. ( f ) Representative images. ( g ) Quantification of the MT intensity around sperm. Box-and-whisker plots show median (horizontal line), interquartile range (box) and maximum/minimum range (whiskers). n >30 structures from three independent experiments. *** P <0.001, **** P <0.0001 (Student’s t -test, two-tailed). Bars, 20 μm. Full size image MEL-28 is needed for chromatin-driven microtubule nucleation MEL-28 is concentrated on kinetochores and might thus primarily function there. To examine this, we assembled spindles around chromatin-coated beads that lack both kinetochores and centrosomes [15] . On MEL-28 depletion, microtubule assembly around chromatin beads was severely inhibited ( Fig. 3a–c ), as for sperm nuclei. No microtubules were nucleated around chromatin beads after 10 min ( Fig. 3a,b ). RanGTP-induced aster and spindle formation [16] was also abolished in the absence of MEL-28 ( Fig. 3d,e ). In contrast, the addition of DMSO to both mock and MEL-28-depleted extracts induced similar numbers of aster-like structures ( Supplementary Fig. 2 ). 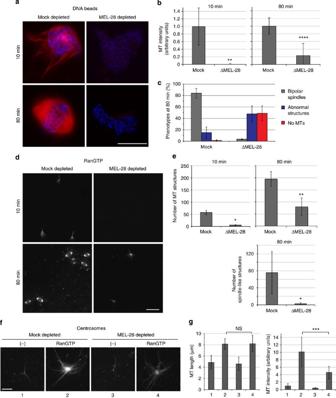Figure 3: MEL-28 is required for RanGTP-dependent microtubule nucleation. (a–c) Chromatin bead spindles were assembled in mock- or MEL-28-depleted CSF extracts. At the indicated time points, aliquots were fixed and spun down on coverslips. (a) Representative images: red, microtubules (MTs); blue, DNA. (b) Quantification of the MT intensity around DNA beads.n>20 DNA bead clusters containing 15–40 beads, which frequently formed bipolar spindles in control extracts. Error bars, s.d. (c) Quantification of spindle phenotypes.n>50 DNA bead clusters. Error bars, s.d. from two experiments. (d,e) RanGTP-mediated MT assembly was examined in control or MEL-28-depleted extracts. Samples were squash-fixed at the indicated time points. (d) Representative MT images. (e) Numbers of MT structures and spindle-like structures were counted in 100 randomly selected fields with a 63 × objective. Error bars, s.d. from four experiments. (f,g) Centrosome-mediated MT assembly was examined in control or MEL-28-depleted extracts. Samples were fixed and spun down on coverslips. Note that this assay was performed in TPX2-depleted extracts that do not nucleate self-organized MTs and allow MT nucleation exclusively from centrosomes. (f) Representative images of asters. (g) MT length and intensity in centrosomal asters were quantified31. n>20 asters. Error bars, s.d. Not significant (NS),P>0.05. *P<0.05, **P<0.01, ***P<0.001, ****P<0.0001 (Student’st-test, two-tailed). Scale bars, 20 μm. Figure 3: MEL-28 is required for RanGTP-dependent microtubule nucleation. ( a – c ) Chromatin bead spindles were assembled in mock- or MEL-28-depleted CSF extracts. At the indicated time points, aliquots were fixed and spun down on coverslips. ( a ) Representative images: red, microtubules (MTs); blue, DNA. ( b ) Quantification of the MT intensity around DNA beads. n >20 DNA bead clusters containing 15–40 beads, which frequently formed bipolar spindles in control extracts. Error bars, s.d. ( c ) Quantification of spindle phenotypes. n >50 DNA bead clusters. Error bars, s.d. from two experiments. ( d , e ) RanGTP-mediated MT assembly was examined in control or MEL-28-depleted extracts. Samples were squash-fixed at the indicated time points. ( d ) Representative MT images. ( e ) Numbers of MT structures and spindle-like structures were counted in 100 randomly selected fields with a 63 × objective. Error bars, s.d. from four experiments. ( f , g ) Centrosome-mediated MT assembly was examined in control or MEL-28-depleted extracts. Samples were fixed and spun down on coverslips. Note that this assay was performed in TPX2-depleted extracts that do not nucleate self-organized MTs and allow MT nucleation exclusively from centrosomes. ( f ) Representative images of asters. ( g ) MT length and intensity in centrosomal asters were quantified [31] . n>20 asters. Error bars, s.d. Not significant (NS), P >0.05. * P <0.05, ** P <0.01, *** P <0.001, **** P <0.0001 (Student’s t -test, two-tailed). Scale bars, 20 μm. Full size image We next analysed whether MEL-28 also regulates microtubule stability. Incubation of centrosomes in control extracts nucleated microtubule asters, and the addition of RanGTP increased microtubule length and density [17] ( Fig. 3f,g ). In MEL-28-depleted extracts, microtubule length increased on RanGTP addition as in the control. In contrast, microtubule intensity was less effectively stimulated by RanGTP ( Fig. 3f,g ). Therefore, MEL-28 is required for RanGTP-dependent microtubule nucleation, but not stabilization. MEL-28 is critical in Ran-dependent recruitment of γ-tubulin RanGTP-dependent microtubule nucleation requires the γ-tubulin ring complex (γTuRC) [18] . Immunoprecipitation of MEL-28 identified γTuRC and Nup107–160 components as main interaction partners ( Fig. 4a ; mass spectrometry in Supplementary Table 2 ). The interaction between MEL-28 and γTuRC was confirmed by γ-tubulin immunoprecipitation ( Fig. 4a ). In contrast, we could not detect interaction between MEL-28 and HURP or TPX2 (ref. 19 ; Fig. 4a ). 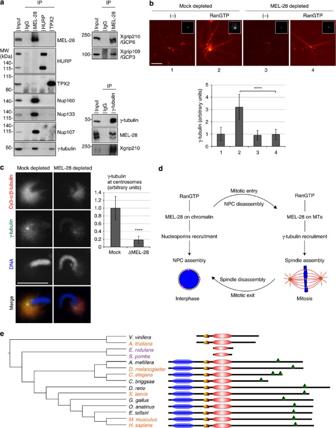Figure 4: MEL-28 is required for RanGTP-dependent recruitment of γ-tubulin. (a) MEL-28 interacts with γTuRC. CSF extract was incubated with protein A beads covalently coupled to control IgG or antibodies against MEL-28, HURP, TPX2 or γ-tubulin. The beads were washed and immunoprecipitates (IP) were analysed by immunoblotting. (b) Centrosomal asters were assembled as inFig. 3f, but subsequently immunostained for γ-tubulin (green). Red, microtubules (MTs). Insets show γ-tubulin signal on centrosomes with the same magnification. Scale bar, 20 μm. γ-Tubulin levels at centrosomes were quantified.n>20 asters. Error bars, s.d. (c) Mock or MEL-28-depleted CSF extracts were incubated with sperm and Cy3-tubulin (red) at 20 °C for 10 min. The samples were fixed, spun down on coverslips and stained for γ-tubulin (green). Scale bar, 20 μm. γ-Tubulin levels at centrosomes were quantified in a 3-μm-diameter circle.n>20 asters assembled around sperm. Error bars, s.d. ****P<0.0001 (Student’st-test, two-tailed). (d) Model to highlight the mutually exclusive functions of MEL-28 to assemble NPCs in interphase or to promote MT nucleation in mitosis (details see text). (e) Domain structure of MEL-28 orthologues. The tree shows the phylogenetic distribution of the selected species according to NCBI taxonomy. Thick black lines indicate the length of each protein. Schematic representation displays β-propeller (blue), coiled-coil domain (yellow), MEL-28/ELYS domain (red) and AT-hook (green). Species known to disassemble NPCs are displayed in orange, and those that keep NPCs assembled during mitosis are in purple (black: no information). Figure 4: MEL-28 is required for RanGTP-dependent recruitment of γ-tubulin. ( a ) MEL-28 interacts with γTuRC. CSF extract was incubated with protein A beads covalently coupled to control IgG or antibodies against MEL-28, HURP, TPX2 or γ-tubulin. The beads were washed and immunoprecipitates (IP) were analysed by immunoblotting. ( b ) Centrosomal asters were assembled as in Fig. 3f , but subsequently immunostained for γ-tubulin (green). Red, microtubules (MTs). Insets show γ-tubulin signal on centrosomes with the same magnification. Scale bar, 20 μm. γ-Tubulin levels at centrosomes were quantified. n >20 asters. Error bars, s.d. ( c ) Mock or MEL-28-depleted CSF extracts were incubated with sperm and Cy3-tubulin (red) at 20 °C for 10 min. The samples were fixed, spun down on coverslips and stained for γ-tubulin (green). Scale bar, 20 μm. γ-Tubulin levels at centrosomes were quantified in a 3-μm-diameter circle. n >20 asters assembled around sperm. Error bars, s.d. **** P <0.0001 (Student’s t -test, two-tailed). ( d ) Model to highlight the mutually exclusive functions of MEL-28 to assemble NPCs in interphase or to promote MT nucleation in mitosis (details see text). ( e ) Domain structure of MEL-28 orthologues. The tree shows the phylogenetic distribution of the selected species according to NCBI taxonomy. Thick black lines indicate the length of each protein. Schematic representation displays β-propeller (blue), coiled-coil domain (yellow), MEL-28/ELYS domain (red) and AT-hook (green). Species known to disassemble NPCs are displayed in orange, and those that keep NPCs assembled during mitosis are in purple (black: no information). Full size image We therefore examined the levels of γ-tubulin on centrosomal asters. RanGTP stimulated γ-tubulin recruitment to centrosomes in control extracts [17] , but not in MEL-28-depleted extracts ( Fig. 4b ). Moreover, γ-tubulin, essential for microtubule nucleation, was recruited to sperm centrosomes at early stages of mitosis in control extracts ( Fig. 4c ) [18] . MEL-28 depletion abolished this recruitment ( Fig. 4c ). These results clearly indicate that MEL-28 binds to microtubules in a RanGTP-dependent manner and recruits γ-tubulin for further microtubule nucleation. Experiments in Xenopus egg extracts showed that at early stages of NPC assembly MEL-28 binds to chromatin in a RanGTP-dependent manner [11] . Chromatin binding is via the C-terminal region containing an AT-hook and an NLS, and is required for the recruitment of other nucleoporins and progression of NPC assembly [20] ( Fig. 4d ). Here we find that on mitotic entry and NPC disassembly, MEL-28 dissociates from chromatin and binds microtubules via the same C-terminal region in a RanGTP-dependent manner ( Fig. 4d ). This allows MEL-28 to play its roles in microtubule assembly and spindle formation. MEL-28 binding to chromatin or microtubules using the same C-terminal region may discriminate its function in interphase and mitosis in a mutually exclusive way. Interestingly, yeast cells undergo mitosis without disassembling NPCs and express ELY5 (35 kD) as an orthologue of metazoan MEL-28 (>200 kD) [21] . ELY5 comprises only the central α-helical MEL-28/ELYS domain and lacks all other domains (β-propeller, coiled-coil and unstructured C-terminal domain containing the AT-hook and the NLS) ( Fig. 4e and Supplementary Fig. 3 ). Yeast ELY5 is a component of NPCs, but, in contrast to metazoans, is not required for NPC assembly [21] . Fungi with the minimal MEL-28 domain also do not disassemble NPCs during mitosis [22] ( Fig. 4e ). Taken together, these data suggest that the RanGTP-dependent functions of MEL-28 in interphase and mitosis evolved with NPC disassembly and open mitosis. MEL-28 is specifically required for RanGTP-dependent microtubule nucleation in egg extract, like TPX2 and HURP [19] . MEL-28, however, does not associate with these two proteins, but interacts with γTuRC and the Nup107–160 complex. MEL-28, TPX2 and HURP may be involved in different steps of RanGTP-dependent microtubule nucleation [23] . TPX2 depletion induces the most severe defects in Ran-induced microtubule nucleation [3] , whereas MEL-28 depletion results in the most severe defects in sperm spindle assembly. We hypothesize that TPX2 is critical for de novo formation of microtubules in the vicinity of chromatin. MEL-28 binds to pre-existing microtubules, nucleated by TPX2 or from centrosomes, in a RanGTP-dependent manner and recruits γ-tubulin to promote additional microtubule nucleation. MEL-28 thus drives positive feedback in RanGTP-mediated microtubule nucleation [24] , [25] . The nearly complete absence of microtubules around chromatin in MEL-28-depleted extracts may be attributable to the chromatin-bound protein Dppa2, which locally inhibits microtubule assembly [26] . Dppa2 on chromatin may effectively depolymerize microtubules nucleated by TPX2 and centrosomes in the absence of MEL-28. In contrast, it hardly affects further amplified microtubules in the presence of MEL-28. γTuRC primarily localizes to centrosomes and spindle microtubules under physiological conditions [18] and accumulates at kinetochores only when microtubule attachments are disrupted [27] . Our data support the idea that MEL-28 primarily functions in microtubule nucleation at the spindle. It has been shown previously that the Nup107–160 complex partially localizes to the spindle and is required for spindle assembly in egg extracts [28] . We provide strong evidence that MEL-28 is the MAP recruiting the Nup107–160 complex and γTuRC to microtubules, and is the key factor for RanGTP-dependent microtubule nucleation. In summary, we have discovered a new role for MEL-28 as a RanGTP-dependent MAP required for microtubule nucleation and spindle assembly. Our data highlight that the cell cycle-dependent association of MEL-28 exclusively drives NPC assembly at the end of mitosis and spindle assembly in early mitosis ( Fig. 4d ). Xenopus egg extracts Cytostatic factor-arrested M-phase Xenopus laevis egg extracts (CSF extracts) were prepared [29] , [30] . Xenopus eggs were dejellied by cysteine treatment, washed with XB buffer (10 mM K–HEPES, 100 mM KCl, 1 mM MgCl 2 , 0.1 mM CaCl 2 and 50 mM sucrose, pH 7.7) and subsequently with CSF–XB buffer (10 mM K–HEPES, 100 mM KCl, 3 mM MgCl 2 , 0.1 mM CaCl 2 , 50 mM sucrose and 5 mM EGTA, pH 7.7) and crushed by centrifugation at 20,000 g for 20 min at 16 °C. The straw-coloured middle layer was recovered as a CSF extract. Endogenous MEL-28 was depleted from CSF extracts by two rounds of incubation with 60% (vol/vol) Dynabeads Protein A (Life Technologies) coupled with Xenopus MEL-28 antibody [11] (0.3 μg antibody applied per 1 μl beads). CSF extracts were supplemented with Cy3-labelled tubulin and incubated with sperm nuclei or chromatin beads for spindle assembly [30] . Microtubule density around sperm or beads was quantified using Matlab (The MathWorks) [31] . For rescue experiments, mRNA encoding Xenopus MEL-28 (GenBank accession KJ026765) was prepared using the mMESSAGE mMachine kit (Life Technologies) and added to extracts at a concentration of 300 ng μl −1 . Recombinant proteins and antibodies For recombinant fragments of Xenopus MEL-28 (KJ026765), cDNAs encoding aa 1,441–2,201 and aa 1,993–2,201 were subcloned into pGEX-6P-1. The GST fusion proteins were expressed in E. coli and purified with Glutathione Sepharose (GE Healthcare Life Sciences). His-tagged aa 1,602–2,120 was expressed in E. coli and purified with Ni-NTA (Qiagen) [11] . His, GFP-tagged aa 1,441–2,201 was constructed in pET28a (Novagen), expressed in E. coli and purified with Ni-NTA and Superose 6 (GE Healthcare Life Sciences). His-importin-α, His-importin-β and His-RanQ69L-GTP were expressed in E. coli and purified with TALON beads (Clontech) [31] . The following published and commercial antibodies were used: Xenopus MEL-28 antibody, human MEL-28 antibody against aa 1,572–2,266, Xenopus 160 antibody [11] , human Nup107, Nup133 and Nup160 antibodies (Abcam ab85916, ab57645 and ab74147, respectively), γ-tubulin antibody from mice (Sigma T6557), γ-tubulin antibody from rabbits [32] , Xgrip109 and 210 antibodies [33] . The human MEL-28 antibody was produced in rabbits against recombinant aa 1,208–1,800, Xenopus Nup107 antibody was produced against aa 1–164 and Xenopus Nup133 antibody was produced against aa 640–1,060. Microtubule assays in vitro and in egg extracts Microtubule sedimentation assay: HeLa nuclear extract (4C Biotech) was diluted with CSF–XB buffer to 1 mg ml −1 and centrifuged at 100,000 g for 10 min at 20 °C. The supernatant was incubated with 2 μM taxol-stabilized microtubules at room temperature (RT) for 15 min in the presence of 1 mM GTP and 10 μM taxol. The samples were centrifuged at 100,000 g for 10 min at 20 °C, and the supernatant and pellet were analysed by SDS–PAGE and immunoblotting. Recombinant MEL-28 fragments were incubated with MTs in the same way but in the presence of 0.05 mg ml −1 BSA. Microscopy-based microtubule-binding assay was performed in vitro [7] . GFP MEL-28 aa 1,441–2,201 (1 μM) was incubated with Cy3-labelled, taxol-stabilized MTs (0.3 μM) at RT for 10 min in BRB80 buffer (80 mM K-PIPES, 1 mM MgCl 2 , 1 mM EGTA, pH6.8) supplemented with 20 μM taxol. The samples were squashed with fixative. The RanGTP-dependent microtubule nucleation assay [16] : CSF extracts were incubated with 15 μM RanQ69L-GTP and 1 μM Cy3-tubulin at 20 °C for 80 min. The samples (Ran spindles and asters) were squashed with fixative. The RanGTP-dependent microtubule stabilization assay [31] : TPX2-depleted CSF extracts were incubated with 1 μM Cy3-tubulin and 2,000 centrosomes per μl in the presence or absence of 15 μM RanQ69L-GTP at 20 °C for 30 min. The samples (centrosomal asters) were fixed and spun down on coverslips. Immunofluorescence CSF extract was supplemented with sperm nuclei and Alexa 488-labelled tubulin, and driven into interphase by adding calcium and incubating at 20 °C for 90 min. Samples were cycled into mitosis by adding a fresh CSF extract and incubating at 20 °C for 80 min. Cy3-labelled Xenopus MEL-28 antibody was added to the extract at a 5 ng μl −1 concentration 10 min before fixation. Interphase nuclei and mitotic spindles were fixed and spun down on coverslips. DNA was stained with Hoechst 33342. HeLa cells were first permeabilized with 0.1% Triton X-100 in PHEM buffer (60 mM PIPES, 20 mM HEPES, pH 6.9, 10 mM EGTA, 4 mM MgSO 4 ) at RT for 5 min and then fixed with −20 °C methanol for 5 min [28] . The cells were stained with human MEL-28 antibody (1 μg ml −1 , against aa 1,572–2,266 or aa 1,208–1,800) and anti-α-tubulin DM1A (1:1,000; Sigma T9026) followed by Alexa 488-labelled anti-rabbit IgG and Alexa 568-labelled anti-mouse IgG (Life Technologies). DNA was stained with Hoechst. Chromatin isolation CSF extract supplemented with sperm and Cy3-tubulin were driven into interphase and cycled into mitosis as described above. At each time point, an aliquot was taken and chromatin was isolated [34] . Samples were diluted with 5 volumes of XB buffer and centrifuged at 5,000 g for 12 min through a 0.7-M sucrose cushion. After removing the supernatant, nuclear pellets were resuspended in XB, 0.3% Triton X-100 and incubated for 5 min on ice. After an additional 10,000 g centrifugation for 2 min, the chromatin fraction (pellet) was recovered. Microscopy Fluorescence images were acquired using a Zeiss Cell Observer microscope, a Plan-Apo 63 × NA 1.4 oil objective, an AxioCam MRm camera and the AxioVision software. Images were also acquired at 0.5-μm Z steps using a Leica SP5 confocal microscope equipped with a 63 × Plan-apochromat NA 1.4 oil-immersion objective. Maximum intensity projections were obtained using ImageJ (NIH). Immunoprecipitations Dynabeads Protein A were coupled with various purified antibodies and cross-linked with dimethyl pimelimidate (Sigma) [35] . Each bead sample (60 μl slurry) was incubated with CSF extracts (100 μl) at 4 °C for 60 min and washed twice with CSF–XB and twice with CSF–XB containing 0.5 M KCl and 0.1% Triton X-100. The immunoprecipitates were separated by SDS–PAGE for immunoblotting. We also analysed control and MEL-28 immunoprecipitates by mass spectrometry [32] . In brief, proteins of the immunoprecipitates were separated by SDS–PAGE, and proteins in-gel were digested by trypsin. Samples were analysed using an ESI LTQ Orbitrap mass spectrometer (Thermo Fisher, Dreieich, Germany). Bioinformatics Homologues of X. laevis MEL-28 were identified with a PSI-BLAST three-iteration search against the non-redundant protein sequences database, performed on the NCBI server ( http://blast.ncbi.nlm.nih.gov/Blast.cgi ) with default parameters. Representative protein sequences were then selected and aligned using T-Coffee with default parameters [36] . The resulting alignment was visualized with Jalview [37] coloured with Clustal X colour scheme. A hidden Markov model was built from the annotated AT-hook sequences using the HHsuite 2.0 package [38] , which was used to identify this DNA-binding domain in other homologous proteins with HHsearch. Secondary structures were predicted by PSIPRED [39] , whereas disorder was predicted with IUPred [40] . The phylogenetic tree was generated with iTOL [41] based on the eukaryotic NCBI taxonomy tree. Western blots Original scans of the cropped images in the main figures ( Figs 1a,e , 2a and 4a ) are presented in Supplementary Fig. 4 . How to cite this article: Yokoyama, H. et al. The nucleoporin MEL-28 promotes RanGTP-dependent γ-tubulin recruitment and microtubule nucleation in mitotic spindle formation. Nat. Commun. 5:3270 doi: 10.1038/ncomms4270 (2014).